Development of oculomotor circuitry independent ofhox3genes Hox genes have been shown to be essential in vertebrate neural circuit formation and their depletion has resulted in homeotic transformations with neuron loss and miswiring. Here we quantifiy four eye movements in the zebrafish mutant valentino and hox3 knockdowns, and find that contrary to the classical model, oculomotor circuits in hindbrain rhombomeres 5–6 develop and function independently of hox3 genes. All subgroups of oculomotor neurons are present, as well as their input and output connections. Ectopic connections are also established, targeting two specific subsets of horizontal neurons, and the resultant novel eye movements coexists with baseline behaviours. We conclude that the high expression of hox3 genes in rhombomeres 5–6 serves to prevent aberrant neuronal identity and behaviours, but does not appear to be necessary for a comprehensive assembly of functional oculomotor circuits. Molecular and anatomical characterizations have been used to study the role of Hox genes in neuronal differentiation and wiring of hindbrain circuits that mediate behaviours such as postural and motor control [1] , [2] , [3] , [4] , [5] , [6] , [7] . Using behavioural (for example, escape response [8] and respiration [9] ) and physiological (calcium imaging [8] and electrophysiology [9] , [10] ) measurements, previous studies have documented the emergence of ectopic neurons and circuits after Hox perturbation. The presence of these neurons has been interpreted as a transformation at rhombomeric levels. In contrast, this study measured the motor output performance of normal circuits, with analyses on ectopic circuits subsequently superimposed. These circuits and this approach allowed comprehensive evaluation of the developmental integrity and functional state of rhombomeres (r). Specifically, the influence of valentino and downstream hox3 genes on r5–6 was investigated by measuring the performance of four normal eye movement behaviours involving different sensory input and motor output. These behavioural performances provided information on the functional state of five neuronal subgroups and their specific connections (>10). This assessment was further complemented with anatomical and genetic analyses, which highlighted the links between genes, development and behaviour in larval zebrafish. Vertebrate eye movements occur in three dimensions ( Fig. 1a–c ), which enables tracking of visual targets and stabilization of gaze with respect to world- or self-motion [11] , [12] . The connectivity and physiological function of individual nuclei comprising the hindbrain circuits generating these oculomotor behaviours have been extensively characterized [13] , [14] , [15] . This neural architecture serves as a platform for superimposing genetic perturbations ( Fig. 1d ). Connections within and outside the hindbrain provide an excellent model to study the influence of genes beyond their restricted hindbrain expression domain ( Fig. 1e ). Horizontal and torsional/vertical eye movements emerge stereotypically in larval zebrafish ( Fig. 1a–c ) [11] , [12] . Quantitative measurements of these behaviours allow simultaneous assessment of multiple neuronal subgroups and connections in vivo and enable a comprehensive characterization of circuit development. 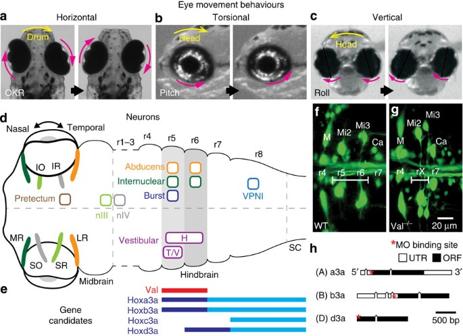Figure 1: Eye movement behaviours with corresponding neuronal and genetic components in larval zebrafish. (a–c) Horizontal (a), torsional (b) and vertical (c) eye movements of a zebrafish larva at 5 dpf. (d) Neurons and extraocular muscles that generate behaviours depicted ina–c. (e) Anterior–posterior expression pattern ofhox3paralogues andvalentino28. (f,g) Retrograde labelling of reticulospinal neurons in wild type (f) andval−/−(g) showing the size reduction of r5–6 inval−/−(rX, bracket). (h) Schematic showing the targeting sites of the three morpholinos used in this study. Ca, caudal zone reticular neuron; H and T/V, horizontal and torsional/vertical vestibular; IO, inferior oblique; IR, inferior rectus; LR, lateral rectus; M, Mauthner cell; Mi 2 and 3, Middle zone reticular neurons; MR, medial rectus; SO; superior oblique; SR, superior rectus; VPNI, velocity-position-neural-integrator. Figure 1: Eye movement behaviours with corresponding neuronal and genetic components in larval zebrafish. ( a – c ) Horizontal ( a ), torsional ( b ) and vertical ( c ) eye movements of a zebrafish larva at 5 dpf. ( d ) Neurons and extraocular muscles that generate behaviours depicted in a – c . ( e ) Anterior–posterior expression pattern of hox3 paralogues and valentino [28] . ( f , g ) Retrograde labelling of reticulospinal neurons in wild type ( f ) and val −/− ( g ) showing the size reduction of r5–6 in val −/− (rX, bracket). ( h ) Schematic showing the targeting sites of the three morpholinos used in this study. Ca, caudal zone reticular neuron; H and T/V, horizontal and torsional/vertical vestibular; IO, inferior oblique; IR, inferior rectus; LR, lateral rectus; M, Mauthner cell; Mi 2 and 3, Middle zone reticular neurons; MR, medial rectus; SO; superior oblique; SR, superior rectus; VPNI, velocity-position-neural-integrator. Full size image The vertebrate hindbrain is subdivided into segments called rhombomeres [16] . Each rhombomere contains a distinct set of neurons that are specified by a network of highly regulated transcription factors [1] , [16] , [17] , [18] . Most of the eye movement neurons and connections are located in r5–6 ( Fig. 1d ) [11] , [19] , [20] , [21] , [22] . Thus, we selected two gene candidates that are strongly expressed in r5–6 and presumed to be essential in the development of the oculomotor circuits: (1) valentino ( val/mafb ), a zebrafish homologue of kreisler in mouse [23] , [24] and (2) hox3 paralogues ( Fig. 1e ) [25] . Val/mafb is expressed in r5–6 and regulates hox3 and eph/ephrin signalling [23] , [24] , [26] , [27] , [28] , [29] , [30] . Both kreisler [31] , [32] and valentino mutants [24] exhibited a diminished r5–6 anterior–posterior dimension (r5–6/rX; Fig. 1f,g ). Molecular characterizations at embryonic stages in both species indicated a lack of abducens motoneurons that are essential for all horizontal eye movements [24] , [32] . In zebrafish there are four hox3 paralogues acting downstream of val/mafb , three of which are expressed in r5–6 ( Fig. 1e and Supplementary Fig. 1 ) [28] , [30] . Hox genes are crucial in defining respiratory neuron projections [33] , assembling auditory circuits [10] and facial motoneuron migration [34] . Specifically, hox3 paralogues have been shown to be necessary for motoneuron specification [35] , [36] , [37] and connectivity [36] , [38] , [39] . Based on these established roles for val/mafb and hox3 , any perturbation of these genes would result in dysfunctional oculomotor circuits and behaviours, if at all present. In this study, oculomotor circuits are functionally assessed in larvae of the val mutant ( Fig. 1g ) and hox3 antisense morpholino knockdowns ( Fig. 1h ). Contrary to predictions, all eye movement behaviours are observed, indicating the existence of all oculomotor subgroups and their correct connections. In some cases, circuit performance is as good as that in wild type, demonstrating oculomotor circuit development is independent from hox3 influence. Unexpectedly, a novel, horizontal ‘saccade-like’ behaviour is also observed with high penetrance in val −/− and phenocopied in hox3 knockdowns. This behaviour is not generated by saccadic burst neurons, but by an ectopic input from a pattern generator synchronized with jaw and fin movements. The targeting of two specific horizontal subnuclei demonstrates that although hox3 genes could be envisioned to play a role in negating neuronal transformations, they do not appear to be necessary for the overall development of oculomotor circuits. Eye movement behaviours By 5 days post fertilization (dpf), larval zebrafish exhibited horizontal ( Fig. 1a ), torsional ( Fig. 1b ) and vertical ( Fig. 1c ) eye movements in response to either visual or vestibular stimuli. The underlying neurons ( Fig. 1d ) and circuits ( Supplementary Figs 2A,B and 3 ) [13] , [40] , [41] served as a template to assess the presence and input/output connectivity of oculomotor neurons. Four oculomotor behaviours were measured and quantified, namely (1) optokinetic reflex (OKR), (2) spontaneous scanning saccades, (3) eye position holding, and (4) torsional and vertical eye movements. These behaviours were first examined in the valentino mutant and then in the knockdown of downstream hox3 paralogues. Optokinetic reflex During horizontal whole-field visual stimulus, zebrafish larvae exhibit an OKR, which minimizes the difference between eye and stimulus velocity [41] . The OKR can be divided into a slow phase for tracking and a fast phase for resetting eye position when the eyes become eccentric in the orbit ( Fig. 2a and Supplementary Fig. 2A,B ). The slow phase can be separated into an early direct component ( Fig. 2a and Supplementary Fig. 2A ), principally reflecting a direct pretectal input, and a subsequent indirect component [42] showing the horizontal vestibular contribution to eye velocity maintenance. Analysis of these behaviours represents the structure and function of four neuronal subgroups located in r5/6 (Vest (H), Burst, Abd and Int; Fig. 2b,c and Supplementary Fig. 2A,B ). 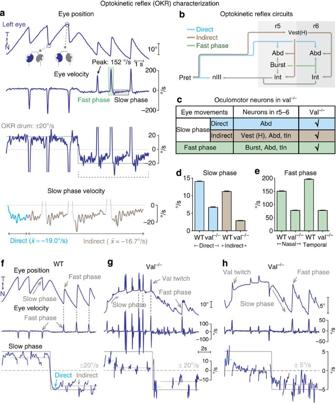Figure 2: Optokinetic reflex behaviour in wild-type andvalentinolarvae. (a) Quantitative and qualitative analyses of OKR. (a) Eye position records were acquired and differentiated into velocity. Fast phase velocity was measured in low gain sweeps. Traces were desaccaded12(dashed bracket) and the slow phase velocity (expanded view) divided into direct and indirect components to quantify performance. (b) OKR can be separated into slow and fast phases that involve specific sets of neurons. Schematic illustrating the circuits for slow and fast phases. Refer toSupplementary Fig. 2for the detailed wiring of the circuits. (c) Table summarizing eye movements observed inval−/−with the neurons in r5–6 highlighted. (d–e) Histograms showing the performance of Slow (d) and Fast phases (e) inval−/−when compared with wild type. Wild-typen: Slow phase (direct=713; indirect=716), fast phase (nasal=950; temporal=939).Val−/−n: Slow phase (direct=972; indirect=1,047), fast phase (nasal=790; temporal=987), error bars (s.e.m.). (f,g) Representative OKR responses for one velocity step cycle of ±20°/s and (h) ±5°/s at 0.0625 Hz in wild type (f) andval−/−(g,h). Blue and brown lines represent mean velocity of direct and indirect components, respectively. Abd, abducens motoneurons; Int, internuclear neurons; nIII, oculomotor nucleus; N, nasal; Pret, pretectum; T, temporal; Vest(H), horizontal vestibular neurons. Figure 2: Optokinetic reflex behaviour in wild-type and valentino larvae. ( a ) Quantitative and qualitative analyses of OKR. ( a ) Eye position records were acquired and differentiated into velocity. Fast phase velocity was measured in low gain sweeps. Traces were desaccaded [12] (dashed bracket) and the slow phase velocity (expanded view) divided into direct and indirect components to quantify performance. ( b ) OKR can be separated into slow and fast phases that involve specific sets of neurons. Schematic illustrating the circuits for slow and fast phases. Refer to Supplementary Fig. 2 for the detailed wiring of the circuits. ( c ) Table summarizing eye movements observed in val −/− with the neurons in r5–6 highlighted. ( d – e ) Histograms showing the performance of Slow ( d ) and Fast phases ( e ) in val −/− when compared with wild type. Wild-type n : Slow phase (direct=713; indirect=716), fast phase (nasal=950; temporal=939). Val −/− n : Slow phase (direct=972; indirect=1,047), fast phase (nasal=790; temporal=987), error bars (s.e.m.). ( f , g ) Representative OKR responses for one velocity step cycle of ±20°/s and ( h ) ±5°/s at 0.0625 Hz in wild type ( f ) and val −/− ( g , h ). Blue and brown lines represent mean velocity of direct and indirect components, respectively. Abd, abducens motoneurons; Int, internuclear neurons; nIII, oculomotor nucleus; N, nasal; Pret, pretectum; T, temporal; Vest(H), horizontal vestibular neurons. Full size image Visual velocity steps (that is, position triangles, Fig. 2a ) were used to quantify OKR behaviour, because this waveform resolves both direct and indirect components of slow phase in addition to fast phase ( Fig. 2a–c ). Wild-type larvae exhibited slow phase tracking in the direction of the stimulus with a direct velocity of 14.04±0.12°/s and indirect component of 11.18±0.17°/s ( Fig. 2d and Supplementary Figs. 2C,D ). Fast phases occurred in the opposite direction with a temporal velocity of 195.5±2.5°/s, larger than the nasal component of 150.2±2.1°/s, ( Fig. 2e and Supplementary Fig. 2E ). Tracking of a ±20°/s stimulus in 5 dpf larvae enabled the comparison of slow and fast phase in wild type and val −/− eye position records ( Fig. 2f–h , arrows). Both behaviours in val −/− often coexisted with a ‘saccade-like’ twitching behaviour hereafter referred to as the ‘val twitch’ ( Supplementary Movie 1 ). Val twitches were independent of eye position and stimulus direction ( Fig. 2g ). The use of a lower step velocity stimulus (5°/s) permitted both slow and fast phase behaviours to be better distinguished in the val −/− eye position records ( Fig. 2g,h ). Close examination of the velocity records at 20°/s ( Fig. 2g ) revealed that val −/− displayed all aspects of OKR, albeit with a general reduction in performance ( Fig. 2g , indirect). Val −/− exhibited a slow-phase direct velocity of 6.18±0.18°/s and an indirect velocity of 2.36±0.12°/s, which were 56% and 79% reduced compared with that of wild type, respectively ( Fig. 2d ). Fast-phase eye velocity was 77.42±1.36°/s in nasal direction and 77.46±1.26°/s in temporal direction, which were 48% and 60% reduced compared with wild type, respectively ( Fig. 2e ). In summary, the presence of horizontal OKR behaviour in val −/− demonstrated the existence of all horizontal neuronal subgroups and circuitry both within and outside r5–6. Spontaneous saccades Spontaneous saccades are produced by burst neurons located in r5. The saccadic circuit architecture [14] , [15] , [19] , [22] is shown in Fig. 3a and Supplementary Fig. 2B . Similar to that in fast-phase resetting behaviour ( Fig. 2c ), the activation of burst neurons during spontaneous saccades results in a rapid eye movement to a new holding position ( Fig. 3b and Supplementary Fig. 2B ). In wild-type larvae, spontaneous saccades occurred both in the presence (light) or absence (dark) of visual input ( Fig. 3c and Supplementary Movie 2 ) [43] . In val −/− , spontaneous eye motion in both light and dark was often dominated by twitches that intermingled with spontaneous saccades ( Fig. 3d ). Spontaneous saccades exhibited an average velocity of 136.6±4.7°/s in wild type and 103.8±6.4°/s in val −/− ( Supplementary Fig. 2 ). Although reduced in frequency and amplitude, the presence of spontaneous scanning saccadic behaviour demonstrated functional burst neuron circuitry. 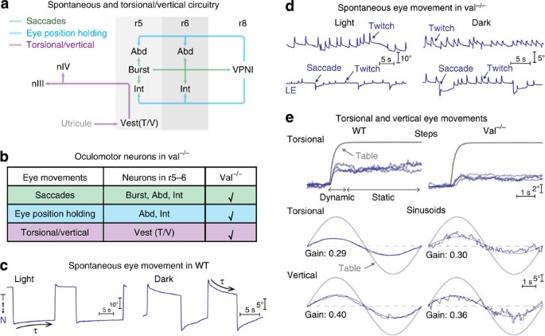Figure 3: Spontaneous scanning saccades with eye position holding and torsional/vertical eye movements. (a) Schematic illustration of the circuits producing the above eye movements.Supplementary Figs 2 and 3show a detailed wiring of the circuits. (b) Table summarizing eye movements observed inval−/−with neurons in r5–6 highlighted. (c,d) Eye position traces showing representative spontaneous eye movements. (c) In light and dark for wild type. (d) In light and dark forval−/−. (e) Representative eye position traces showing torsional and vertical eye movements in wild type andval−/−. Torsional responses to position steps and sinusoids. Vertical responses to a sinusoidal stimulus. Although present in only the horizontal plane, val twitches (Supplementary Movie 2) were picked up by the algorithm and represented by the dashed lines. Figure 3: Spontaneous scanning saccades with eye position holding and torsional/vertical eye movements. ( a ) Schematic illustration of the circuits producing the above eye movements. Supplementary Figs 2 and 3 show a detailed wiring of the circuits. ( b ) Table summarizing eye movements observed in val −/− with neurons in r5–6 highlighted. ( c , d ) Eye position traces showing representative spontaneous eye movements. ( c ) In light and dark for wild type. ( d ) In light and dark for val −/− . ( e ) Representative eye position traces showing torsional and vertical eye movements in wild type and val −/− . Torsional responses to position steps and sinusoids. Vertical responses to a sinusoidal stimulus. Although present in only the horizontal plane, val twitches ( Supplementary Movie 2 ) were picked up by the algorithm and represented by the dashed lines. Full size image Eye position holding After spontaneous saccades, the ability to maintain an eccentric eye position in the light is supported by visual feedback ( Fig. 2b , pretectal input) and by a velocity-to-position neural integration (see Fig. 3a and Supplementary Fig. 2A for VPNI (Velocity-position-neural-integrator) circuitry). In the dark, eye position holding is only supported by VPNI [43] , [44] , [45] , [46] , [47] whose functional state and connections with Abd/Int neurons in r5–6 can be quantified with a decay time constant ( τ ) [44] , [45] , [48] ( Fig. 3c , arrows). This time constant is always greater in the presence of visual feedback than in the dark [43] . In val −/− , spontaneous saccades were observed, often with twitches superimposed ( Fig. 3d ). The time constant of the spontaneous saccades in val −/− was 2.26±0.49 s ( n =19) and lay within the size related range of 1.5–5.0 s reported previously in wild-type larvae [49] . In summary, the presence of eye position holding in val −/− demonstrated the existence of a functional input from r5 burst neurons to r8 VPNI neurons, and then to r5–6 Abd/Int neurons ( Fig. 3a ). Torsional and vertical eye movements In response to head and/or body displacements in three-dimensional space, zebrafish larvae produce compensatory torsional and vertical eye movements for gaze stabilization [11] . These eye movements are mediated by topographical projections from utricular afferents onto two principal neuronal types in the tangential nucleus in r5 (Vest(T/V)) [11] , [50] . Different sets of extraocular muscles are controlled to produce compensatory eye rotations along the pitch and roll axes [11] ( Figs 1b,c and 3a,b ; detailed architecture in Supplementary Fig. 3 ). Compensatory torsional and vertical eye movements in val −/− larvae were observed in response to position steps ( Fig. 3e ) and sinusoidal ( Fig. 3e ) changes in head position. Twitches were only observed in the horizontal, but not in torsional or vertical, eye movements ( Supplementary Movie 2 ). As compared with wild-type siblings, val −/− larvae exhibited an ~40% decrease in amplitude of the dynamic/static components for a pitch tilt step from 0° to 10° ( Fig. 3e ). The torsional and vertical responses to sinusoidal stimuli were reduced and highly variable between val −/− larvae, but in some cases both gains could be comparable to wild-type siblings ( Fig. 3e and Supplementary Movie 2 ). These results showed functional vestibular circuitry in val −/− that required the presence of a r5-specific tangential nucleus. Behaviour summary In summary, all four oculomotor behaviours were found in val −/− . These four behaviours demonstrated the existence of horizontal vestibular, tangential, burst, abducens and internuclear neurons in r5–6 of val −/− . This included their functional connections with areas outside of r5–6 (forebrain pretectum, midbrain oculomotor nucleus (nIII), trochlear nucleus (nIV) in r1, VPNI in r8 and the vestibular ganglion as illustrated in Figs 1d , 2b and 3a ). The twitches were only observed during horizontal and not vertical and torsional eye movement behaviours. Abducens motoneurons in valentino Previous studies using molecular markers claimed the absence of Abd in val −/− [24] , [51] ; however, the presence of temporal eye movement produced by the lateral rectus muscle during OKR and spontaneous saccades ( Figs 2a and 3c , and Supplementary Figs 2A and B ) strongly argued for the presence of Abd motoneurons. For confirmation, florescent dye was placed in the orbit [11] to identify Abd Mns in r5–6 ( Fig. 4a,b ). To visualize both the Abd Mns and VIth nerve, an olig2 enhancer-trap line [19] was used in which Abd and oligodendrocyte precursors were genetically labelled with the florescent protein kaede. In both control ( Fig. 4c,e ) and val −/− ( Fig. 4d,f ), Abd Mns (circles) were observed at the same anterior–posterior level of the otic vesicles (r5) and their axons formed the VIth nerve (white and red arrows in Fig. 4c,d and Fig. 4e,f , respectively). As it is impossible to definitively distinguish Abd from olig2 + oligodendrocyte precursors, the diameter of the VIth nerve when it exits the brain was used as a proxy for the number of Abd neurons and was used to compare the size of the Abd nucleus in val −/− and control. In val −/− , the diameter of the VIth nerve averaged 5.64±0.37 μm ( n =12) and was similar ( P =0.32; t -test) to 4.89±0.34 μm in wild-type siblings ( n =5). Therefore, given the similarities in eye abduction performance and diameter of the VIth nerve, the Abd nucleus exists in valentino mutant and is likely to have similar size as in wild type. 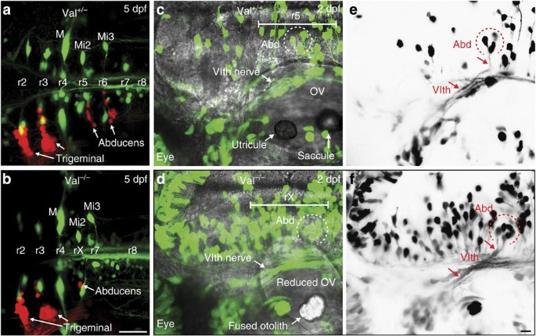Figure 4: Abducens motoneurons inval−/−. (a,b) Retrograde labelling from the orbit (red) visualized both abducens and trigeminal motoneurons in 5 dpfval+/−(a) andval−/−(b). Rhombomeres were identified by recticulospinal neurons (M, Mi2 and Mi3) back-filled from the spinal cord (green). (c,d) VIth nerve of 2 dpfval+/−(c) andval−/−(d) were visualized in the Gal4s1020tolig2kaede enhancer-trap line. (e,f) Projections of selected confocal planes of fromcandd, respectively, in which VIth nerve axons can be traced back to Abd cell body. The neurons shown are a partial representation of the whole abducens nucleus. Scale bars, 50 μm (a,b) and 10 μm (c,d). Figure 4: Abducens motoneurons in val −/− . ( a , b ) Retrograde labelling from the orbit (red) visualized both abducens and trigeminal motoneurons in 5 dpf val +/− ( a ) and val −/− ( b ). Rhombomeres were identified by recticulospinal neurons (M, Mi2 and Mi3) back-filled from the spinal cord (green). ( c , d ) VIth nerve of 2 dpf val +/− ( c ) and val −/− ( d ) were visualized in the Gal4s1020t olig2 kaede enhancer-trap line. ( e , f ) Projections of selected confocal planes of from c and d , respectively, in which VIth nerve axons can be traced back to Abd cell body. The neurons shown are a partial representation of the whole abducens nucleus. Scale bars, 50 μm ( a , b ) and 10 μm ( c , d ). Full size image Properties of Val twitches Eye position decay time constants ( τ ) of intermingled spontaneous saccades and twitches were 2.2 and 0.2 s, respectively ( Fig. 5a ). The val twitch τ dark of 0.12±0.02 s ( n =147) was approximately two orders of magnitude lower than that of 9.46±0.9 s for spontaneous saccades in wild type ( n =65; Fig. 5b ). The val twitch τ light of 0.10±0.01 s ( n =217) was similar to τ dark ( Fig. 5c ), indicating the absence of visual feedback during the behaviour, unlike in wild-type saccades ( Fig. 5b ). In val −/− , all possible combinations of twitches were observed in the four monocular horizontal circuits (for example, left versus right eye, nasal (N) versus temporal (T); Figs 3d and 5d,f ). These quantitative findings demonstrated twitches were not produced by burst, VPNI or vestibular pathways, and suggested that an ectopic input connects solely with Abd Mns and Int neurons. 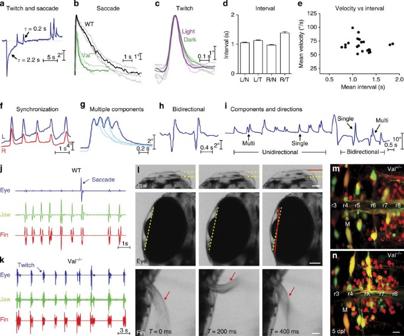Figure 5: Properties of val twitches. (a) Eye position traces inval−/−showing the co-existence of twitches and spontaneous saccades with differentτ. (b) Overlay of eye position traces following spontaneous saccade inval−/−(green) and wild type (black). (c) Representative eye position traces of twitches in light (purple) and dark (green) showing similar decay time constants. (d) Intervals between left (L) and right (R) nasal (N), and left and right temporal (T) twitches were ~1 s (n=1,827 from 14 larvae), Error bars in s.e.m. (e) Plot of twitch velocity versus twitch interval showing no correlation (r2=0.04;n=21). (f) Synchronized twitches between left and right eye. (g) Multiple components within individual twitch episodes. (h) Bidirectional twitches that involved both lateral and medial rectus muscles. (i) A representative eye position trace showing twitches with uni-/bimodal and single/multiple components combinations. (j,k) Normalized acceleration profiles of the eye, lower jaw and fin movements. (j) Spontaneous fin and jaw movements were time-locked, but eye movements were independent in wild type. (k) Eye twitches inval−/−were time-locked to lower jaw and fin movements. (l) Still images from a high-speed recording (100 Hz) showing the relative temporal onset for eye, jaw and fin movement. Yellow dashed and red solid lines mark the original and new position of the jaws and eye, respectively. (m,n) Sequential retrograde labelling visualizing reticular neurons that project only to the anterior spinal cord (red only) in (m)val+/−(n=9) and (n)val−/−(n=11). Scale bars, 10 μm. Figure 5: Properties of val twitches. ( a ) Eye position traces in val −/− showing the co-existence of twitches and spontaneous saccades with different τ . ( b ) Overlay of eye position traces following spontaneous saccade in val −/− (green) and wild type (black). ( c ) Representative eye position traces of twitches in light (purple) and dark (green) showing similar decay time constants. ( d ) Intervals between left (L) and right (R) nasal (N), and left and right temporal (T) twitches were ~1 s ( n =1,827 from 14 larvae), Error bars in s.e.m. ( e ) Plot of twitch velocity versus twitch interval showing no correlation ( r 2 =0.04; n =21). ( f ) Synchronized twitches between left and right eye. ( g ) Multiple components within individual twitch episodes. ( h ) Bidirectional twitches that involved both lateral and medial rectus muscles. ( i ) A representative eye position trace showing twitches with uni-/bimodal and single/multiple components combinations. ( j , k ) Normalized acceleration profiles of the eye, lower jaw and fin movements. ( j ) Spontaneous fin and jaw movements were time-locked, but eye movements were independent in wild type. ( k ) Eye twitches in val −/− were time-locked to lower jaw and fin movements. ( l ) Still images from a high-speed recording (100 Hz) showing the relative temporal onset for eye, jaw and fin movement. Yellow dashed and red solid lines mark the original and new position of the jaws and eye, respectively. ( m , n ) Sequential retrograde labelling visualizing reticular neurons that project only to the anterior spinal cord (red only) in ( m ) val +/− ( n =9) and ( n ) val −/− ( n =11). Scale bars, 10 μm. Full size image The twitches exhibited a velocity of 67.6±2.2°/s ( Supplementary Fig. 2F ), lower than the saccadic velocity of 136.6±4.7°/s and 103.8±6.4°/s in wild type and val −/− , respectively. The difference in twitch and saccadic velocities along with the difference in τ dark indicated that spontaneous saccade and twitch generations were independent. In addition, twitch velocities were similar regardless of the presence or absence of coexisting saccades ( Supplementary Fig. 2F ), suggesting that the twitches were generated independently from the r5 burst neurons [14] , [15] , [19] . The mean intervals between twitches in all four monocular circuits were consistently around 1 s (between 0.97 and 1.38 s; Fig. 5d ). Regression analysis of the intervals with velocity showed no correlation ( Fig. 5e ). Therefore, a twitch pattern generator (tPG) with an unidentified location operated at ~1 Hz and mediated the timing of twitches, but not the velocity. Single-component twitches were the most typical ( Fig. 5f ), but episodes exhibiting multiple components (up to four; Fig. 5g ) suggested repetitive triggering tPG bursts. Twitches appeared in either the temporal or nasal direction (unidirectional, Fig. 5f,g ) or as two closely timed twitches in the same eye in opposite directions (bidirectional, Fig. 5h ). When both eyes exhibited twitches, the events were synchronized ( Fig. 5f ) irrespective of which extraocular muscle was involved, suggesting a common upstream tPG. Ectopic connections could be made to both Abd and Int neurons independently and generate uni-/bidirectional twitches occurring in any combination in the same larva ( Fig. 5i ), illustrating the stochastic nature of this tPG-mediated behaviour. Correlation with jaw and fin The val twitches were temporally correlated with jaw/operculum openings and fin movements ( Fig. 5k,l and Supplementary Movie 3 ). In wild type, spontaneous jaw and fin movements were synchronous ( Fig. 5j and Supplementary Movie 3 ) and spontaneous saccades were often time-locked, but not rhythmically coupled to the jaw/fin movement ( Fig. 5j , saccade arrow). In contrast, eye twitches in val −/− were always time-locked with each episode of jaw/fin movement ( Fig. 5k , twitch arrow). Analysis of high-speed video recordings ( Fig. 5l ) revealed the jaw and eye movements were synchronous ( n =38; P =0.254, t -test). However, pectoral fin movements led the eye/jaw movements by 112.7±9.2 ms ( n =38; P <0.0001, t -test) ( Fig. 5l , Supplementary Fig. 4A–C and Supplementary Movie 3 ). Time-locking suggested the tPG linking spontaneous jaw and fin movement was also generating the horizontal twitches. Sequential retrograde labelling from two spinal sites of the reticular spinal scaffold distinguished neurons projecting only to the rostral spinal cord. The majority of these reticular neurons were located in r7–8 in control larvae (red only neurons in Fig. 5m ), regardless of the efficacy of the labelling technique. In val −/− , an increased number of neurons exhibited such projection patterns in r5–6 (or rX) ( Fig. 5n ). These observations demonstrated neuronal projection of r5–6 neurons in val −/− was more r7–8-like and may be permissive for the establishment of ectopic connections such as those generating val twitches. Oculomotor circuitry in val −/− Horizontal oculomotor behaviours in val −/− , although present, were generally less robust ( Fig. 2d–f ). Twitches were often superimposed on horizontal oculomotor behaviours ( Figs 2f , 3d and 5a ), suggesting the underlying circuits were functional. Two lines of evidence indicated the horizontal oculomotor circuitry was present and functional in valentino . First, oculomotor performance switched between a ‘twitch’ and ‘normal’ mode in val −/− ( Fig. 6a–e ). Val twitches appeared to override normal oculomotor behaviours; however, when absent, episodes of wild-type-like horizontal eye movement were observed ( Fig. 6a–e ). In Fig. 6a , the left eye medial rectus exhibited twitches and OKR tracking gain was 0.35 ( Fig. 6b ). Three minutes later, a normal mode appeared with OKR tracking gains of 0.8 ( Fig. 6c ) and 0.69 ( Fig. 6d ), typical for wild-type larvae when presented with similar stimuli. In normal mode epochs, this val −/− larva produced spontaneous saccades with τ dark of 13.51±4.87 s ( n =5; Fig. 6e ). After 28 min, the val −/− larva switched back to a twitch mode and displayed robust, spontaneous val twitches ( Fig. 6e ). These results demonstrated the presence of a nearly normal horizontal circuitry in val −/− that was intermittently masked by the tPG twitches. 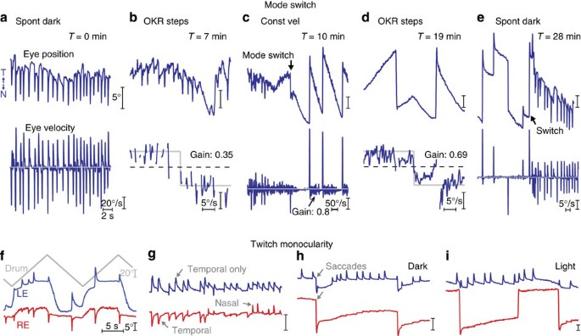Figure 6: Mode switch and characterization of the ectopic input inval−/−. Example of switching inval−/−between a ‘twitch’ (a,b) and a ‘normal’ mode (c–e). OKR performance and spontaneous saccades during normal mode inc–ewere similar to wild type. OKR stimuli were ±5°/s steps (b,d) and 5°/s constant velocity (e). (f–i) Observed variations in ectopic input. (f) Val twitches superimposed on OKR behaviours in both eyes. (g) Val twitches in different sets of muscles in each eye. (h,i) Twitches in only the left eye while the right eye showed wild-type-like behaviours. Twitches superimposed on the spontaneous saccades in the dark (h) or light (i). Figure 6: Mode switch and characterization of the ectopic input in val −/− . Example of switching in val −/− between a ‘twitch’ ( a , b ) and a ‘normal’ mode ( c – e ). OKR performance and spontaneous saccades during normal mode in c – e were similar to wild type. OKR stimuli were ±5°/s steps ( b , d ) and 5°/s constant velocity ( e ). ( f – i ) Observed variations in ectopic input. ( f ) Val twitches superimposed on OKR behaviours in both eyes. ( g ) Val twitches in different sets of muscles in each eye. ( h , i ) Twitches in only the left eye while the right eye showed wild-type-like behaviours. Twitches superimposed on the spontaneous saccades in the dark ( h ) or light ( i ). Full size image Val twitches often involved both the left and right eye, with independent recruitment of lateral rectus and medial rectus ( Figs 5f and 6f,g ). However, there were cases when only one eye exhibited twitches (left eye in Fig. 6h,i ), while the other eye behaved normally ( Fig. 6h,i ). These data demonstrated the ectopic tPG could target circuits monocularly with the unaffected circuit remaining fully functional. Together, these findings showed that the horizontal circuits developed normally, established essential connections and could perform at a wild-type level in val −/− even in the presence of ectopic input from a tPG. Hox3 knockdown phenocopies twitch behaviour Val/mfab is upstream of eph/ephrin and hox3 signalling [23] , [24] , [26] , [27] , [28] , [29] , [30] . Given the documented roles of hox3 genes in establishing r5–6-specific neuronal identity and circuit wiring [35] , [36] , [37] , [38] , [39] , their absence could permit the generation of ectopic twitch connections observed in val −/− . To test this hypothesis, hox3 genes were knocked down using antisense morpholinos and oculomotor behaviours were quantified at 5 dpf. Three out of the four hox3 paralogues were expressed in r5–6 in zebrafish ( Fig. 1e ) with the exception of hoxc3a ( Supplementary Fig. 1 ) [28] . The val twitch phenotype was found in 66.7% of 12 larvae that received a combination of 4, 2 and 2 ng for hoxa3a , b3a and d3a morpholinos, respectively. Other combinations of hox3 paralogues in 24 larvae did not reproduce the phenotype ( Supplementary Fig. 5A,B ). Oculomotor behaviours of the hox3 morphants were qualitatively similar to those observed val −/− ( Fig. 7a ). The morphants exhibited OKR slow phase tracking with both direct and indirect components ( Fig. 7b ), fast-phase resets (arrows in Fig. 7b ) and twitches ( Fig. 7b ). In this case only the left eye (blue trace) exhibited twitches while the right eye (red trace) performed OKR similar to wild type. Quantification of the behaviours showed that all OKR measurements (slow and fast phase components) were reduced compared with control ( Fig. 7c,d and Supplementary Fig. 2C–E ). Spontaneous scanning eye movements were observed with an eye position holding decay time constant of 5.86±0.96 s ( n =37). The decay time constant for twitches of 0.125±0.002 s ( n =137; Fig. 7e ) was similar to that in val −/− (0.12±0.02 s; Fig. 7e ). Switching between ‘normal’ and ‘twitch’ modes was also observed ( Fig. 7e ). 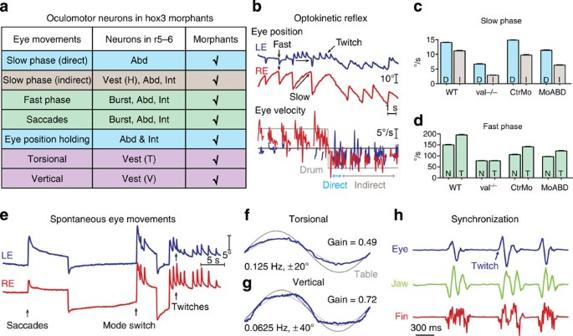Figure 7: Eye movement behaviours inhox3morphants. (a) Table summarizing the eye movement neurons in r5–6 and behaviours observed inhox3morphants that phenocopied the val twitch. (b) Eye position and velocity traces during OKR showing the presence of slow phases exhibiting both direct and indirect components, fast phases and superimposed val twitches. (c,d) Quantification of slow (c) and fast (d) phase eye velocities showing a reduced performance in morphants when compared with either control morphants or wild type, but less so than inval−/−. Slow phasen: direct=478; indirect=483. Fast phasen: nasal=711; temporal=775, Error bars in s.e.m. (e) A representative eye position trace showing the presence of spontaneous saccades, eye position holding, mode switch and synchronized twitches. (f) Torsional and (g) vertical vestibulo–ocular reflex (VOR) of morphants (n=5). (h) Synchronization of jaw and pectoral fin movements with eye twitches. Figure 7: Eye movement behaviours in hox3 morphants. ( a ) Table summarizing the eye movement neurons in r5–6 and behaviours observed in hox3 morphants that phenocopied the val twitch. ( b ) Eye position and velocity traces during OKR showing the presence of slow phases exhibiting both direct and indirect components, fast phases and superimposed val twitches. ( c , d ) Quantification of slow ( c ) and fast ( d ) phase eye velocities showing a reduced performance in morphants when compared with either control morphants or wild type, but less so than in val −/− . Slow phase n : direct=478; indirect=483. Fast phase n : nasal=711; temporal=775, Error bars in s.e.m. ( e ) A representative eye position trace showing the presence of spontaneous saccades, eye position holding, mode switch and synchronized twitches. ( f ) Torsional and ( g ) vertical vestibulo–ocular reflex (VOR) of morphants ( n =5). ( h ) Synchronization of jaw and pectoral fin movements with eye twitches. Full size image Torsional and vertical eye movements were particularly robust in hox3 morphants ( Fig. 7f,g ). Torsional eye movement performance in hox3 morphants exhibited gains of ~0.5 over a wide frequency range. The performance was better than in val −/− and similar to that reported in wild type [11] ( Supplementary Fig. 5C ). As in val −/− , twitches in the morphants were only observed in horizontal, but not torsional or vertical, eye movements. High-speed video showed that twitches in morphants were also time locked to jaw and fin movements ( Fig. 7h ). Retrograde labelling of reticular spinal scaffold demonstrated a normal sized r5/6 as opposed to the much-reduced r5/6 in val −/− ( Supplementary Fig. 5D,E ). This observation implies that the later was a consequence of defective eph/ephrin signalling and independent of hox3 (ref. 26 ). Surprisingly, there were no obvious alterations in cellular morphology and location of identified reticular neurons ( Supplementary Fig. 5E ). In summary, knockdown of hox3 alone showed that development of the horizontal and vertical oculomotor circuits was independent of all three hox3 paralogues in r5–6. The presence of twitch behaviours reinforced the idea that hox3 genes are responsible for preventing the aberrant connections to Abd Mns and Int neurons. Our study demonstrated hox3 genes were not essential for oculomotor circuit development. In val −/− , the predominant hox3 expression in r5–6 was non-existent [28] . Classical views would predict homeotic transformation of these rhombomeres and thus a nearly complete loss of r5–6-specific neurons and their corresponding behaviours [1] , [7] , [18] . This study provided four unequivocal lines of evidence showing this prediction does not apply to the hox3 paralogous group and oculomotor circuits: (1) behavioural data showed that all r5–6 nuclei related to horizontal eye movements acquired their specific identities, established functional connections and produced oculomotor behaviours in the val mutant and hox3 knockdowns ( Figs. 2 , 3 and 7 ). (2) The vestibulo–ocular reflex pathway for torsional and vertical eye movements developed in the absence of hox3 genes and produced compensatory behaviours, indicating the presence of topographical projections that extended from the sensory periphery to the r5-specific tangential nucleus ( Figs 3 and 7 ) [11] , [50] . (3) At a cellular level, genetic, anatomical and functional evidence demonstrated the presence of abducens motoneurons that were previously reported to be absent ( Figs. 2 , 3 , 4 ) [24] . (4) Irrespective of rhombomeric morphology and/or size, in particular the extreme case of val −/− where r5–6 were highly reduced in size, all oculomotor performances could be comparable to wild type, especially in the absence of val twitches (mode switch; Fig. 6 ). Thus, the underlying circuitry exhibited a physiological profile adequate to produce wild-type-like oculomotor behaviours. In summary, although hox3 genes have been envisioned to be crucial in r5–6 motoneuron specification and connectivity [35] , [36] , [37] , [38] , [39] , our data demonstrated that development and wiring of the oculomotor circuitry were independent from the entire paralogous hox3 group. Circuit assembly was recently examined in the mammalian auditory system [10] . Mutants of single hox1 or hox2 paralogues exhibited abnormal neuronal specification and pathfinding, as well as impaired hearing, suggesting a decisive role of these Hox genes in all stages of auditory circuit formation [10] . By contrast, our study investigated the role of Hox genes during assembly of the oculomotor circuitry and demonstrated the absence of hox3 had minimal influence on the identity and connectivity of oculomotor neurons resident in r5–6. Horizontal, vertical and torsional eye tracking, as well as eye-holding behaviours, dependent on r5/6 neurons and circuits, were present in both val −/− and hox3 morphants. These behaviours were present in larvae that exhibited either a diminished or a grossly normal rhombomeric structure. The apparent neuron loss in val −/− , which exhibited a reduced r5–6 anterior–posterior dimension (rX), did not preclude the formation of functional eye movement circuitry. Only horizontal eye movement behaviour was intermittently degraded by the activity of an ectopic circuit associated with the knockdown of hox3 . The contrasting level of Hox influence on neuronal identity and circuit formation in the auditory and oculomotor systems illustrates that the role of Hox genes in the hindbrain must be understood and interpreted on a case-by-case basis [3] , [18] , [36] , [52] , [53] . Although not required in oculomotor circuit development, hox3 paralogues played a role in precluding aberrant r5–6 connections. In the absence of hox3 , an ectopic input to the horizontal circuit (specific to Abd and Int neurons) generated a novel, saccade-like twitch behaviour with a high penetrance in val −/− that was phenocopied by hox3 knockdown ( Figs 2 , 3 and 7 ). Lower jaw and operculum opening forces water across the gills for respiration in zebrafish [54] . Meanwhile, fin movement in larval zebrafish has been proposed to enhance respiration by fluid mixing [55] . Twitches were time locked to lower jaw/operculum and fin movements ( Figs 5k and 7h ). Therefore, the tPG is temporally correlated, and maybe linked, to a respiratory pattern generator ( Figs 5k and 8a ). 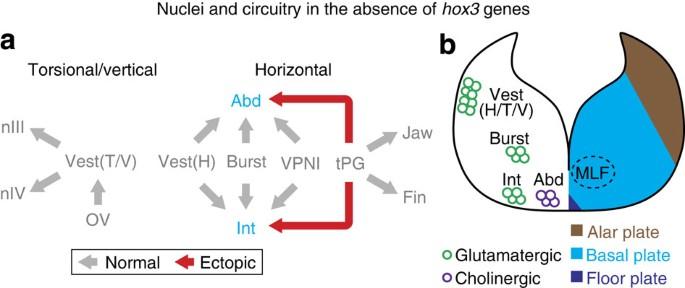Figure 8: Summary comparison of neurons and circuits in the presence and absence ofhox3genes. (a) Schematic showing circuit- and nucleus-specific requirement ofHox3genes in the hindbrain. Only Abd and Int neurons of the horizontal circuit (blue) received the ectopic connections (in red) in the absence of a normal r5–6 Hox3 environment (red arrow). Normal connections (grey arrows) of the horizontal and torsional/vertical circuits were unaffected. (b) A schematic coronal section of r5–6 showing the different embryonic origins and neurotransmitter phenotypes of the identified oculomotor neurons inval−/−andhox3knockdowns. Figure 8: Summary comparison of neurons and circuits in the presence and absence of hox3 genes. ( a ) Schematic showing circuit- and nucleus-specific requirement of Hox3 genes in the hindbrain. Only Abd and Int neurons of the horizontal circuit (blue) received the ectopic connections (in red) in the absence of a normal r5–6 Hox3 environment (red arrow). Normal connections (grey arrows) of the horizontal and torsional/vertical circuits were unaffected. ( b ) A schematic coronal section of r5–6 showing the different embryonic origins and neurotransmitter phenotypes of the identified oculomotor neurons in val −/− and hox3 knockdowns. Full size image By ruling out three potential oculomotor subnuclei, our results suggested ectopic connections existed solely between the tPG and abducens motor/internuclear neurons. Neither VPNI neurons in r8 nor burst neurons in r5 could be the targets because activation of either subgroup would result in eye position holding ( Fig. 3a–c and Supplementary Fig. 2 ) that would be inconsistent with the observed short twitch decay time constants ( Fig. 5c ). In addition, horizontal vestibular neurons were not involved because the time-to-peak and decay in eye position of val twitches were identical in either light or dark ( Fig. 5c ). These observations also showed that pretectal visual input was not part of the twitch circuit. Therefore, we conclude that the ectopic connection generating val twitches existed exclusively between the tPG and Abd motor/Int neurons. Twitches could be either uni- or bidirectional, demonstrating that Abd Mns and Int neurons were targeted independently, and likely to be randomly, by subsets of neurons from the tPG ( Figs 5f–I and 6f–i ). Collectively, these data revealed that hox3 genes act in a nucleus-specific manner. In this case, their influence was limited to the Abd Mns and Int neurons but not in the other subsets of r5–6 neurons, such as burst or vestibular (H, T/V) neurons ( Fig. 8a ). Such restrictions to specific subnuclei in r5–6 are further illustrated in Fig. 8b , which shows ectopic connections only targeted two subsets of basal plate-derived neurons exhibiting different neurotransmitter phenotypes (cholinergic Abd and glutamatergic Int), but not other neurons that share the same origin and/or neurotransmitter phenotype (for example, glutamatergic burst or vestibular neurons) [21] , [22] , [56] , [57] , [58] . Such specificity may arise from differential spatial and/or temporal activities of hox3 paralogues in individual nuclei as previously observed with single hox4 paralogues [59] . For example, hox3 genes may suppress the expression of a secreted guidance cue protein that attracts axons of the tPG neurons. Such a role might explain the continued expression of Hox genes beyond embryonic stages, followed by a downregulation as the circuits mature [7] , [59] . In summary, hox3 genes played a role in preventing extraneous wiring of horizontal Abd Mns and Int neurons in r5–6. Our data has described, for the first time, a partial homeosis at a nucleus level. Abd Mns and Int neurons received ectopic tPG input in the absence of hox3 genes and produced val twitches that coexist with normal oculomotor behaviours ( Figs 2 , 3 , 5 and 6 ). In val −/− and hox3 knockdowns, the rhythmical twitches were generally the observed behaviour; however, when twitches were temporarily absent, functional horizontal eye movement circuits with wild-type-level optokinetic tracking and eye position resets were observed (mode switch in Figs 6a–e and 7e ). Such wild-type-level behavioural performance indicated the abducens nuclei received inputs from vestibular, burst and VPNI neurons with well-differentiated membrane properties suited to produce correct motor output in the absence of hox3 ( Fig. 8a ). Anatomical and genetic assessments using the marker olig2 keade further corroborated the presence of Abd nucleus and VIth nerve ( Fig. 4 ). Superimposition of twitches on the normal behaviours ( Figs 2g,h , 3d and 6f-i ) demonstrated that the tPG input terminated directly onto the Abd subnuclei that were already endowed with a proper set of oculomotor connections, thereby demonstrating a partial homeosis of Abd Mns and Int neurons. These results were not expected because previous loss-of-function studies after Hox perturbations had observed transformed neurons and connections to replace natural circuit functions [2] , [3] , [4] , [5] , [6] , [9] , [10] . Synchronicity among val twitches, jaw and fin movements ( Fig. 5k,l ) suggested the pattern generator responsible for twitches to be most probably located in r8. In zebrafish, pectoral fin movements are produced by motoneurons located in caudal r8 and the anterior spinal cord [60] . Lower jaw movements involve trigeminal (r2–3 nV), facial (r6–7 nVII) [61] and hypobranchial motoneurons (r8) [60] with respiration-correlated neurons principally observed in r8 (ref. 47 ). Therefore, hindbrain r8 appears to be a leading common site for these motor behaviours and thus the ostensible location of the tPG that specifically targets r5–6 Abd Mns and Int neurons in the absence of hox3 . Previous studies suggested r5–6 in val −/− were transformed into a single, reduced segment (rX) with the absence of Abd motoneurons [24] , [51] ; however, our molecular, anatomical and behavioural evidence demonstrated the existence r5-specific neurons including burst and tangential neurons in val −/− ( Figs. 2 , 3 , 4 ). Based on the presence and function of these oculomotor neurons, we concluded that both r5 and r6 (rather then previously proposed rX [24] ) are present despite the reduced anterior–posterior dimension. This interpretation of the r5–6 organization is consistent with data from the mouse mutant kriesler [31] . Conventionally, the repertoire of neurons in a rhombomere after Hox perturbation has been explained by homeosis and/or a redundant activity of other Hox genes and their cofactors [3] , [8] , [52] , [62] . Specific combinations of Hox genes, the ‘Hox code’, have been proposed to determine neuronal identity and connectivity patterns [18] , [53] . In our study where the entire hox3 paralogous group was affected, neither of these mechanisms would fully explain the presence of five distinct r5–6 neuronal subgroups, as well as their specific sets of pre- and post-synaptic connections. Thus, a more probable interpretation is that the development and wiring of the oculomotor circuit is independent from hox3 . Hox genes have been proposed to be key players in neural circuit evolution [18] , [60] . The previously mentioned auditory circuits in mice exhibited connections with the cochlea, a mammalian-only end organ [63] . The observed Hox dependence [63] could represent an evolutionary transformation correlating with increased circuit complexity. By contrast, the horizontal and torsional/vertical vestibulo–ocular and optokinetic circuitry in fish have a lengthy evolutionary history, traceable to agnatha (jawless fish) [64] , [65] , [66] . Reference frames of these circuits, namely head and visual motions, remained unchanged from agnatha to actinopterygian (such as zebrafish) [67] . The relative independence oculomotor circuits acquired from hox3 genes may have contributed to their stability throughout evolution. The coexistence of natural and novel connections observed in this study emphasized the modular organization of neuronal circuits. Through Hox expression modification, previously unrelated circuit modules can be rewired to generate novel behaviours. This rewiring represents a conceivable mechanism for existing neurons and circuits to evolve novel function. Animals Animal handling and experimental procedures were approved by the Institutional Animal Care and Use Committee of New York University School of Medicine (New York, NY). Fish lines were maintained in a centralized facility following standard protocols. Fish lines AB , Et(-0.6hsp70l:Gal4-VP16)s1020t/+;Tg(UAS-E1b:Kaede)s1999t/+ ( Gal4s1020t ) and mafba b377/+ ( valentino ) was obtained from the Zebrafish International Resource Center. The Isl1-GFP line was a kind gift from the Fetcho group in Cornell, NY. Morpholinos Antisense morpholino oligos were obtained from Gene Tools, LLC (Philomath, OR). Two translation blocking ( hoxa3a (5′-CGTCGCAGTAGGTTGCCTTTTGCAT-3′); hoxd3a (5′-TGTCATAATAAGTGGCTTTCTGCAT-3′)), one splice blocking ( hoxb3a 5′-CTGACCTGAAAGGTTATAAGAGGCA-3′) and the Random control oligo (25-base random sequence mixture) morpholinos were used in this study. Morpholino were injected into at one- to two-cell stage using combinations and doses listed in Supplementary Fig. 5 . The efficacy of hoxb3a knockdown was measured by PCR analysis in 2 dpf hoxb3a morphants using the primer set 5′-GAAGGGCACTTGAAGACAAC-3′ (forward) and 5′-TGTACTTCATCCGCCTGTTC-3′ (reverse). All morphants were morphologically normal, except the inability to inflate their swim bladders ( n =56) based on conventional criteria including normal body length, absence of abnormal cell death, normal eye size and response to touch and tap. Behavioural analyses Eye movement behaviours were analysed at 5 dpf in hox3 morphants or larvae from crosses of heterozygous valentino . Horizontal (at 200 Hz), torsional (at 50 Hz) and vertical (at 50 Hz) eye movements were measured in zebrafish immobilized in a block of low-temperature melting agarose (2.0%; Sigma Type VII-A) [11] , [12] . The agarose was removed from around the mouth, jaws and eyes to the level of the otic vesicle and the block affixed with pins to a Sylgard 182 (Dow Corning, Midland, MI) template submerged in 30% Danieau’s solution (17.4 mM NaCl, 0.21 mM KCl, 0.12 mM MgSO 4 ·7H 2 O, 0.18 mM Ca(NO 3 ) 2 and 1.5 mM HEPES (pH 7.2)) and placed in a 25-mm glass cube for torsional and vertical, and 19-mm diameter glass cylinder for horizontal eye movement experiment. Spontaneous eye movement and responses to either optokinetic or vestibular stimuli were recorded with a custom-written algorithm in LabView (National Instrument). OKR were invoked by a drum with alternating black and white stripes (each stripe subtended 15.5°) rotating at either ±5°/s or ±20°/s. Both velocity step and sinusoidal waveforms were employed at 0.0625 Hz. The slow phase response for each half cycle of the OKR stimulus period was separated into a direct component (0–1.5 s but with amplitude measurement from 0 crossing) and indirect component (1.5–7.5 s). Vestibuloocular reflexes were produced by either 10° position steps from +60° to −60° or sinusoids with maximum velocity of 15.7°/s over a frequency range of 0.0625–2 Hz. Mean eye velocity during slow phases (direct and indirect), fast phases and saccades were calculated using algorithms written in Matlab. Eye position holding time constants were determined by exponential fits of eye position traces selected from 500 ms after and 200 ms before saccades [12] . Owing to the brevity of twitches, the entire waveform from peak to baseline was fit for the decay time constant. High-speed videos were recorded using a Pike IEEE 1394b camera (Allied Vision Technology) with a custom-written algorithm in LabView. Data were analysed using Excel (Microsoft), Prism (Graphpad) and Matlab (Mathworks). All larvae from heterozygous valentino crosses were subjected to PCR genotyping using the primer set 5′-CAGCCCCACAGAACAGAAGAACC-3′ (forward) and 5′-ACAAGCTGGTCGTCGGAGAAGC-3′ (reverse), followed by restriction fragment length polymorphism assay using the restriction enzyme Pvu II. Heat shock Larvae of crosses between Gal4s1020t/val −/+ were heated shocked three times at 38 °C for 40 min with 2.5-h intervals starting at 36 hpf [68] . Under this protocol, abducens motoneurons (including their axons) and oligodendrocyte precursors were labelled [19] . Confocal analyses of olig2-kaede containing neurons were performed between 48 and 50 hpf, after which the larvae were subjected to genotyping as described above. Retrograde labelling Reticulospinal neurons were retrograded labelled using crystals of either Alexa Fluor 488 or 647 10 k dextran (Invitrogen) as previously described [59] . Extraocular and trigeminal motoneurons were labelled by placing Alexa Fluor crystals in the orbital space with a tungsten needle [11] . For sequential retrograde labelling of hindbrain reticular neurons, AF488 crystals were first placed in a spinal lesion at the level of myotome 15 at 4 dpf, followed by a similar labelling with AF 647 at the level of myotome 5 at 5 dpf. All confocal analyses were performed on a LSM 510 system (Carl Zeiss). How to cite this article: Ma, L.-H. et al . Development of oculomotor circuitry independent of hox3 genes. Nat. Commun. 5:4221 doi: 10.1038/ncomms5221 (2014).